Molecular dynamics of single-particle impacts predicts phase diagrams for large scale pattern formation Energetic particle irradiation can cause surface ultra-smoothening, self-organized nanoscale pattern formation or degradation of the structural integrity of nuclear reactor components. A fundamental understanding of the mechanisms governing the selection among these outcomes has been elusive. Here we predict the mechanism governing the transition from pattern formation to flatness using only parameter-free molecular dynamics simulations of single-ion impacts as input into a multiscale analysis, obtaining good agreement with experiment. Our results overturn the paradigm attributing these phenomena to the removal of target atoms via sputter erosion: the mechanism dominating both stability and instability is the impact-induced redistribution of target atoms that are not sputtered away, with erosive effects being essentially irrelevant. We discuss the potential implications for the formation of a mysterious nanoscale topography, leading to surface degradation, of tungsten plasma-facing fusion reactor walls. Consideration of impact-induced redistribution processes may lead to a new design criterion for stability under irradiation. Solids irradiated by energetic beams can, depending on environmental parameters, undergo either surface ultra-smoothening [1] or self-organized nanoscale pattern formation [2] ; the desirability of the latter outcome depends on the context. On the one hand, observations of periodic patterns including high-aspect ratio quantum dots [3] , with occasional long-range order [4] and characteristic spacing, as small as 7 nm (ref. 5 ), have stimulated interest in self-organized pattern formation as a means of sub-lithographic nanofabrication [6] . On the other hand, extended exposure to energetic particle irradiation can lead to the structural degradation of fission and fusion reactor components [7] , [8] . Hence, it is important to be able to predict the expected behaviour within a given environment. Unfortunately, precisely which physical effects cause observed transitions between different regimes [9] , [10] has remained a matter of speculation [11] . At particle energies between 10 2 and 10 4 eV, the irradiation process is dominated by the nuclear collision cascade caused by impact [12] , [13] . Displaced atoms that reach the surface with enough kinetic energy to leave are permanently sputtered away; all other displaced atoms come to rest within the solid or on the surface after phonon emission times of ∼ 10 −12 s. These processes contribute prompt erosive [14] , [15] and prompt redistributive [11] , [16] , [17] components of morphology evolution and are collectively denoted P [ x ]. For most materials other than elemental metals, the damage resulting from accumulated impacts quickly ( ∼ 10 −3 s) leads to the amorphization of a thin layer of target material. Over much longer time scales ( ∼ 100 s), mass transport within this layer by kinetic relaxation processes causes a gradual relaxational effect [14] , [18] . Hence, to the prompt term P [ x ] we add a phenomenological term for the gradual relaxation regime denoted G [ x ], assuming a mechanism of ion-enhanced viscous flow, which is expected to predominate in irradiated amorphous materials near room temperature [18] . The prompt and gradual contributions to the rate of motion of the surface in the normal direction v n then superpose: The prompt regime may be characterized using molecular dynamics (MD) simulations [17] , [19] or experimental methods [20] . Given data from many impact events, we may obtain the 'crater function' Δ h ( x − x ′, θ ) describing the average change in local surface height at a point x resulting from a single-ion impact at x ′, with incidence angle θ (a potential dependence on the surface shape, which is very difficult to capture with MD, is left for future work). We then upscale the crater function into a continuum partial differential equation (PDE) for the surface evolution using a multiscale framework. The theoretical formalism for this process is described in more detail in the Supplementary Information and in ref. 21 ; here we provide a brief summary of the important points for the linear case. Given the crater function Δ h and the flux distribution I ( x ), we write the prompt contribution to surface evolution as a flux-weighted integral of the crater function [11] , [22] : A well-known observation in the field is that scale of the craters is much smaller than the scale of the resulting pattern and of the flux distribution. To exploit this fact, we use a formal multiple-scale analysis, based on a small parameter ɛ related to the ratio of impact scale to pattern scale. This formalism allows ready separation of the spatial dependence of the crater shape (fast) from that of the pattern (slow), and leads eventually to an upscaled description of the prompt regime in moment form: Here the ∇ s represent surface divergences, and the (increasing-order) tensors M ( i ) are simply the angle-dependent moments of the crater function Δ h . Pattern-forming predictions are obtained by linearizing equation (1), and examining the stability of the linearization as a function of the laboratory incidence angle θ . The linearization process follows that given in ref. 14 , and in an appropriate frame of reference one finds that the magnitude of infinitesimal perturbations h away from a flat surface evolve, to leading order in ɛ , according to the PDE where the angle-dependent coefficients are determined from the first moments obtained using MD, and the constant coefficient B is estimated from independent experiments. The structure of equation (4) indicates that linear stability is determined strictly by the signs of the calculated coefficients ( S X , S Y ): for values of θ where either of these coefficients is negative, linearly unstable modes exist and we expect patterns, whereas for values of θ where they are both positive we expect flat, stable surfaces. Phase diagram prediction To turn equation (4) into a prediction, it is necessary to obtain the angle-dependent moment M (1) . Using MD simulations of single impacts, we collected angle-dependent moments for Si irradiated by Ar + ions at both 100 and 250 eV (the zeroeth moment M (0) , which is propotional to the number of atoms sputtered per ion, was also obtained). 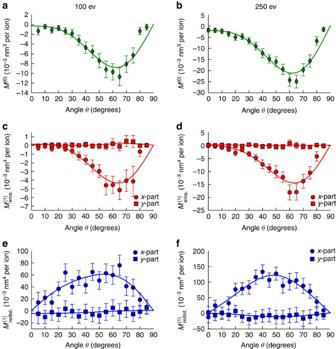Figure 1: Moments obtained from molecular dynamics. Fitted average angle-dependent moments of the crater function Δh(x,y) as determined from molecular dynamics, for both 100 eV (left column) and 250 eV (right column). Error bars indicate a standard 95% confidence interval (±1.96 s.d.) associated with the 200 simulations at each angle. (a,b) Zeroeth erosive momentM(0)(sputter yield times atomic volume). (c,d) First erosive momentsM(1)erosive. (e,f) First redistributive momentsM(1)redist.. Each of the first moments contains components in both the downbeam or 'x'-direction (circles), and also the crossbeam or 'y'-direction (squares), with the crossbeam components expected to be zero from symmetry arguments21. At both energies, redistribution strongly dominates erosion. For each energy, 200 ion impacts were simulated at incidence angles in 5° increments between 0° and 90°, yielding average moments as summarized in Figure 1 . For use within our analytical framework, we fit these moments to Fourier series constrained by symmetry conditions and by the observation that all moments tend to zero at θ =±90°. Finally, the moments were separated into redistributive and erosive components: contributions from displaced atoms coming to rest within or on the solid, and contributions from atoms permanently sputtered away, respectively. For both energies, the redistributive first moments are much larger in magnitude than—and have the opposite sign of—their erosive counterparts. The implication, and main finding of this work, is that redistributive effects completely dominate erosive effects, except possibly at the highest (grazing) angles where all moments tend to zero. Figure 1: Moments obtained from molecular dynamics. Fitted average angle-dependent moments of the crater function Δ h ( x , y ) as determined from molecular dynamics, for both 100 eV (left column) and 250 eV (right column). Error bars indicate a standard 95% confidence interval (±1.96 s.d.) associated with the 200 simulations at each angle. ( a , b ) Zeroeth erosive moment M (0) (sputter yield times atomic volume). ( c , d ) First erosive moments M (1) erosive . ( e , f ) First redistributive moments M (1) redist. . Each of the first moments contains components in both the downbeam or ' x '-direction (circles), and also the crossbeam or ' y '-direction (squares), with the crossbeam components expected to be zero from symmetry arguments [21] . At both energies, redistribution strongly dominates erosion. 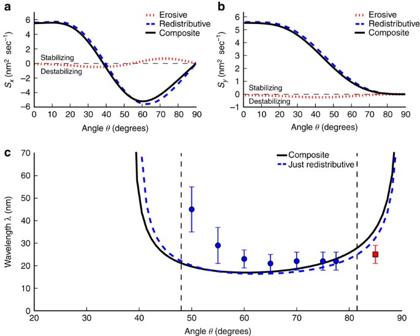Figure 2: Predictions and comparison with experiment. Comparison between predicted and measured wavelength for Si irradiated by Ar+at 250 eV. CoefficientsSX(θ) andSY(θ) in the linearized evolution equation (4) were calculated with a flux off=3.5×1015ions cm−2s−1for comparison with experimental conditions23. (a,b) Coefficients of ∂2h/∂x2and ∂2h/∂y2in the linearized evolution equation using the experimental flux. These coefficients are dominated by redistributive effects. (c) Comparison of predicted ripple wavelengths with average experimentally observed wavelengths (see ref.23). Circles/squares indicate experimental patterns with wavevector parallel/perpendicular to the beam (parallel mode and perpendicular mode, respectively), and the vertical dashed black lines indicate experimental phase boundaries. Error bars indicate the full-width at half-maximum measure of the peaks in the power spectral density associated with atomic force microscopy images of experimental samples. On top of this, the solid black line indicates our predicted wavelengths (which are all parallel mode), and the dashed blue line indicates the wavelengths predicted if erosion were neglected entirely. Full size image Comparison with experiment To corroborate this finding, we calculate in Figure 2 the coefficients (5) of the linearized equation (4) for the 250 eV moments, and compare the pattern wavelengths they predict to experimental observations in the same environmental conditions [23] . (Note: Clean linear experimental data at 100 eV are not currently available. Also, the ripples originally reported in ref. 23 at 250 eV for angles below 20° have been omitted because those authors have recently shown them to be an experimental artefact.) The agreement is excellent, with two minor exceptions. First, the small quantitative difference between predicted and observed phase boundaries—which depends only on the shape of S X ( θ )—could readily arise from the approximate nature of the classical potential, on which our simulations are based (unlike the phase boundary, precise wavelength values depend on the value of B , which could only be estimated). Second, the measured moments do not predict a transition to perpendicular modes at the highest angles; this could be due to our neglect of explicit curvature dependence in the crater function, but additional physical effects such as shadowing and surface channeling—not addressed here—are known to be important at grazing angles. Despite these limitations of our approach, when one considers the lack of any free parameters in the theory, the agreement with experiment is remarkably good. The agreement remains good even when the erosive coefficients are omitted, and the similar shapes of the redistributive moments at 100 and 250 eV is consistent with the reported [23] energy insensitivity of the stability/instability phase boundary. Figure 2: Predictions and comparison with experiment. Comparison between predicted and measured wavelength for Si irradiated by Ar + at 250 eV. Coefficients S X (θ) and S Y (θ) in the linearized evolution equation (4) were calculated with a flux of f =3.5×10 15 ions cm −2 s −1 for comparison with experimental conditions [23] . ( a , b ) Coefficients of ∂ 2 h/ ∂ x 2 and ∂ 2 h/ ∂ y 2 in the linearized evolution equation using the experimental flux. These coefficients are dominated by redistributive effects. ( c ) Comparison of predicted ripple wavelengths with average experimentally observed wavelengths (see ref. 23 ). Circles/squares indicate experimental patterns with wavevector parallel/perpendicular to the beam (parallel mode and perpendicular mode, respectively), and the vertical dashed black lines indicate experimental phase boundaries. Error bars indicate the full-width at half-maximum measure of the peaks in the power spectral density associated with atomic force microscopy images of experimental samples. On top of this, the solid black line indicates our predicted wavelengths (which are all parallel mode), and the dashed blue line indicates the wavelengths predicted if erosion were neglected entirely. Full size image Existing uses of MD crater data for investigations of surface pattern-forming are entirely numerical in nature [24] , and could be viewed as a scheme for numerically integrating equation (2). In contrast, our analytical upscaling of equation (2) into the moment form (3) is notable for several reasons. First, it illustrates exactly which qualities of the crater—namely, its moments—have the dominant role in surface evolution. Second, the moment form can be linearized, allowing predictions of stability boundaries, and changes to those boundaries as crater shape is varied. Third, moments are readily obtainable directly by MD simulation, and converge with far fewer trials than do descriptions of the entire crater function used in previous works. Last, although atomistic methods have been used in the past to obtain the amplitude of a single term in a PDE obtained by phenomenological modelling [17] , [25] , [26] , [27] , we believe this is the first derivation of an entire PDE from MD results. A crucial component of our approach is that the crater function Δ h —and hence the moments M ( i ) —contains the contributions of both erosion and mass redistribution. Whereas these effects have traditionally been treated separately by unrelated phenomenological models, viewing the crater function as fundamental integrates erosion and redistribution into a unified description, allowing both processes to be treated identically and readily separated and compared. Indeed, this approach has permitted us to confirm for the first time conjectures [11] , [19] , [22] that the stability of irradiated surfaces could be dominated by redistributive effects. The most striking aspect of this result is the logical conclusion that erosion is essentially irrelevant for determining the patterns: according to Figure 2 the contributions of redistribution to the S coefficients, which determine stability and patterns, are about an order of magnitude greater and opposite in sign. This conclusion overturns the erosion-based paradigm that has dominated the field for two decades [14] and we suggest its replacement with a redistribution-based paradigm. An important direction for future research is identifying the range of irradiation energies over which our conclusion holds. Because the scale of the impact increases with the energy, higher energies require larger simulation targets, increasing the computational cost of MD simulations. However, preliminary investigations of silicon irradiated by argon at 1 keV, at selected angles spanning the experimental transition point, are so far consistent with our conclusions, and experimental results at 1 keV lead to the same conclusion [28] . As this energy is typical of pattern-forming investigations within the literature, we conclude that it remains to be determined whether erosion is actually important for stability or pattern formation in any physical experiment to date. We believe the phenomena reported in this paper are applicable to a wide variety of systems. For instance, our predictions may be relevant in the context of tungsten plasma-facing fusion reactor walls, in which low-sputter yield (atoms removed per incident particle) has been an important design criterion in the selection of tungsten for surfaces that must be exposed to large plasma particle fluxes for extended periods. Because the average helium ion energy is only ∼ 60 eV and the threshold energy for sputter removal of tungsten is ∼ 100 eV, this material has been considered impervious to the effects of erosion. However, despite a sputter erosion rate that is essentially zero, plasma-facing tungsten, nevertheless, develops under some conditions a nanoscale topography leading to surface degradation [8] —an outcome that appears mysterious within the erosion-based paradigm. The crater function-based analysis presented here suggests that such degradation may originate in impact-induced target atom redistribution effects. A re-analysis of the simulations performed in ref. 29 on helium-irradiated tungsten shows that, after 4,000 consecutive impacts at 100 eV from an incidence angle of 25°, a cumulative displacement field emerges with a clear downbeam bias ( Fig. 3 ). This suggests a redistributive moment that may produce the same stability properties as for those measured above. If this conjecture turns out to be correct, then an extremely low-sputter erosion rate would be an insufficient design criterion for morphologically stable solid surfaces under energetic particle irradiation, and ultimately crater function engineering considerations may provide a more refined materials design criterion. 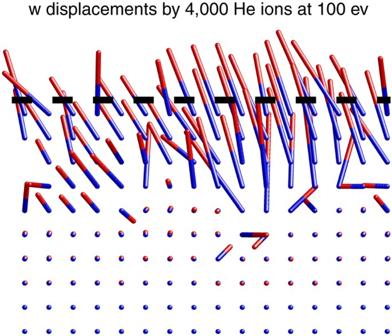Figure 3: Downbeam displacements in helium-irradiated tungsten. Inside a fusion reactor, He irradiates the W walls at low energies (of order 100 eV), generating essentially zero sputter erosion and very little displacement, complicating the isolation within an MD simulation of a clear average signal. However, the cumulative displacement field after 4,000 consecutive off-normal impacts at 100 eV shows a clear downbeam bias. Here impinging helium ions come from the upper right, at an angle of 25° from normal. The sticks combine the initial and final position of atoms that were initially in a half a unit cell thick cross-section through the simulation cell. The blue ends of the sticks indicate the initial positions and the red ends the final positions of the atoms. The surface is located at the top (from a re-analysis of data in ref.29). Figure 3: Downbeam displacements in helium-irradiated tungsten. Inside a fusion reactor, He irradiates the W walls at low energies (of order 100 eV), generating essentially zero sputter erosion and very little displacement, complicating the isolation within an MD simulation of a clear average signal. However, the cumulative displacement field after 4,000 consecutive off-normal impacts at 100 eV shows a clear downbeam bias. Here impinging helium ions come from the upper right, at an angle of 25° from normal. The sticks combine the initial and final position of atoms that were initially in a half a unit cell thick cross-section through the simulation cell. The blue ends of the sticks indicate the initial positions and the red ends the final positions of the atoms. The surface is located at the top (from a re-analysis of data in ref. 29 ). Full size image Simulation environment Our MD simulation environment consists of an amorphous, 20×20×10 nm 3 Si target consisting of 219,488 atoms, with slab boundary conditions (free boundary in the incoming ion direction, and periodic boundaries in the other two lateral directions) [30] . The target itself was created using the Wooten/Winer/Weaire method [31] . Because this method is computationally expensive for large targets, we first constructed a smaller 10×10×10 nm 3 block, and then copied it four times to achieve the desired size. The resulting composite was then annealed with the environment-dependent interatomic potential [32] . This gives an optimized amorphous structure with realistic density, and in which most of the Si atoms have coordination number 4. The target was then bombarded with Ar + at 100 and 250 eV at different incidence angles, with random impact points and azimuthal angles, at an ambient temperature of 0 K. During bombardment, the interaction between Si atoms was again described using the environment-dependent interatomic potential, which gives a good agreement between simulated and experimental sputtering yields [33] , whereas the Ar–Si interaction was a potential calculated for the Ar–Si dimer [34] . Kinetic energy was gradually removed during the simulations from 1 nm borders of the cell to prevent it from re-entering the impact area via the periodic boundary conditions used in the simulations. The simulation arrangements and their suitability for cluster and ion bombardment simulations are discussed in more detail in refs 33 , 35 , 36 , 37 . Obtaining moments For each impact, simulations totalling 15 ps were run, which was enough time for atomic motion to settle to the level of thermal vibration. Final atomic positions were then obtained by averaging the atomic positions for a further 5 ps. Before analysis, this set of post-impact atomic positions was adjusted in two important ways. First, the global average displacement of each atom over all impacts at a given incidence angle was subtracted from its post-impact position for each impact at that angle, to remove target-specific effects from our measurements (see Supplementary Fig. S1 ). Second, an observed shear of the entire target in the downbeam direction—caused by the finite target size—was fitted from data near the bottom of the target, and also subtracted from the post-impact positions (see Supplementary Fig. S2 ). From the initial and adjusted final atomic positions, moments were obtained by assuming that densities in the amorphous layer must attain a steady state over time [21] . Consequently, we project defect distributions immediately to the target surface for the purpose of quantifying crater functions. Within this scheme, the effects of erosion and redistribution are readily separated. Erosive moments are obtained by assigning a height loss at each location proportional to the number of sputtered atoms originating from that location. Similarly, redistributive moments were obtained by assigning height losses at initial atomic positions and height gains at final atomic positions. This strategy produced the data points in Figure 1; the data were then fitted to simple three-term Fourier series to generate the curves in the same figure. Additional details of our simulation environment are available in the Supplementary Information . How to cite this article: Norris, S. A. et al . Molecular dynamics of single-particle impacts predicts phase diagrams for large scale pattern formation. Nat. Commun. 2:276 doi: 10.1038/ncomms1280 (2011).